Fano interference governs wave transport in disordered systems Light localization in disordered systems and Bragg scattering in regular periodic structures are considered traditionally as two entirely opposite phenomena: disorder leads to degradation of coherent Bragg scattering whereas Anderson localization is suppressed by periodicity. Here we reveal a non-trivial link between these two phenomena, through the Fano interference between Bragg scattering and disorder-induced scattering, that triggers both localization and de-localization in random systems. We find unexpected transmission enhancement and spectrum inversion when the Bragg stop-bands are transformed into the Bragg pass-bands solely owing to disorder. Fano resonances are always associated with coherent scattering in regular systems, but our discovery of disorder-induced Fano resonances may provide novel insights into many features of the transport phenomena of photons, phonons, and electrons. Owning to ergodicity, the Fano resonance is a fingerprint feature for any realization of the structure with a certain degree of disorder. Wave transport in perfect periodic systems is described by the propagating Bloch modes that originate from coherent Bragg scattering. However, many periodic structures fabricated these days suffer from inevitable dissimilarity between their structural components. This causes additional disorder-induced destructive scattering. As a result, the wave transport in disordered systems is dominated by random multiple scattering, and the wave propagation can be totally suppressed. Such Anderson localization is universal to all wave systems, and it became a very attractive phenomenon for fundamental demonstrations in optics [1] , [2] , [3] and cold atomic gases [4] , [5] . Anderson localization can be both enhanced and suppressed in certain cases. The combination of the Bragg scattering and disorder is believed to enhance localization of waves in periodic systems. A number of effects may quench the localization [6] , [7] , [8] , [9] and, for example, extended 'necklace states' are possible at certain frequencies [10] , [11] . However, the general mechanisms of an interplay between the order and disorder remain mostly unclear, especially far away from the regime of the Anderson localization. Here we reveal an unexpected link between ordered and disordered systems through a Fano interference [12] , [13] , [14] between periodicity-induced wave propagation and disorder-induced scattering. One of the immediate surprising effects we observe is the switching of the wave transport regime from localization to delocalization by increasing disorder. This leads to unusual transformation of the stop-bands to pass-bands and vice versa, with an asymmetric Fano line-shape observed in between, and it takes place in the specific spectral ranges in the vicinity of the narrow Bragg resonances. Contrary to a common belief and even physical intuition, the interference between various multiple scattering pathways, prerequisite to Fano resonances, does survive the disorder. We believe that this finding may revise our knowledge of transport in disordered systems, since both localization enhancement and suppression occur in the same system, and thus the general physical picture is more complicated and interesting than expected. Our results hold for many systems with a certain type of disorder: electromagnetic waves in photonic crystals with disorder in permittivity, acoustic waves in phononic crystals with randomized density distribution, electrons in semiconductors with fluctuating effective mass. Our general conclusions are supported by both numerical studies and analytical theory. As an example, not restricting generality of our analysis, we study the light propagation in a one-dimensional (1D) photonic crystal described by a simple binary structure ABAB .... Properties of such 1D superlattices have been discussed in many theoretical and experimental studies, [15] including the analysis of the degradation of the photonic bandgaps and enhanced localization in the presence of disorder. [16] , [17] , [18] , [19] , [20] , [21] However, a complete understanding of an interplay between periodicity and Bragg scattering in disordered photonic crystals is still missing. Below, we present a general picture of light localization and de-localization for the case of 1D disordered periodic structures based on numerical studies and analytic theory. Importantly, our results can be compared with the studies of more complicated three-dimensional (3D) structures: synthetic opals [22] , already known for the studies of the effect of disorder on optical spectra [23] , [24] , [25] , [26] , [27] . In opals, the reversal of Bragg bands and transformation of stop-bands into pass-bands were observed experimentally [22] . Inversion of the photonic bandgap spectra A summary of the main effects uncovered below is presented in Fig. 1 . We study the scattering of electromagnetic waves at normal incidence by a stack of alternating A and B layers ( Fig. 1a ) by employing the conventional transfer matrix technique [28] . We assume that the layer widths w A and w B and permittivity ɛ A of the layers A are constant, whereas the layers B introduce disorder with random permittivity characterized by normal distribution around the mean value with the dispersion , and fluctuations in different B layers are uncorrelated. We restrict our analysis by small dielectric contrast . It is well known that almost all modes in (infinite) 1D disordered system become localized, [7] when the disorder is uncorrelated. The transmission coefficient T tends to zero when the number of pairs of layers N increases for all frequencies but a set with measure zero [29] , [30] , [31] . Light transport should be then characterized not by the transmission coefficient itself, but with its decay rate in the limit N →∞. This rate is the extinction χ , defined as T =exp(− Naχ ), where a = w A + w B . In our study, we average the extinction over an ensemble with M disorder realizations. Logarithmic-averaged transmission spectra are then determined from the averaged extinction. Extinction, equivalent to the inverse localization length, is an ergodic self-averaging measure of localization [29] , independent of the structure length and given disorder realization. Because of the self-averaging property, extinction fluctuations are suppressed in long structures. Extinction may be equivalently obtained without ensemble averaging as −lim N →∞ ln T ( N )/ Na . This limit always exists and is nonzero in the whole spectral range excepting possible discrete frequencies [29] . 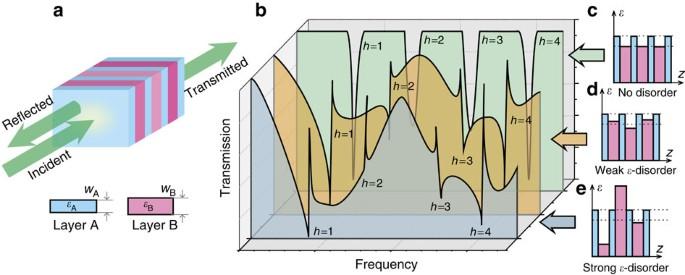Figure 1: Transmission spectra of ordered and disordered photonic crystal structures. (a) Schematic of the 1D photonic crystal and the scattering geometry. The basic parameters of the two layers A and B are:ɛA,wAandɛB,wB. (b) Schematic of typical averaged transmission spectra for ordered periodic structure and for the two structures with fluctuating permittivity. The spectra are shown for the interval of four lower order Bragg bands,h. Corresponding spatial profiles of permittivity of the dielectric layers are shown from the right for (c) no disorder, (d) weakɛ-disorder, and (e) strongɛ-disorder. Figure 1: Transmission spectra of ordered and disordered photonic crystal structures. ( a ) Schematic of the 1D photonic crystal and the scattering geometry. The basic parameters of the two layers A and B are: ɛ A , w A and ɛ B , w B . ( b ) Schematic of typical averaged transmission spectra for ordered periodic structure and for the two structures with fluctuating permittivity. The spectra are shown for the interval of four lower order Bragg bands, h . Corresponding spatial profiles of permittivity of the dielectric layers are shown from the right for ( c ) no disorder, ( d ) weak ɛ -disorder, and ( e ) strong ɛ -disorder. Full size image The transmission spectrum of a perfect photonic crystal (PhC) structure ( , Fig. 1b,c ) consists of narrow equidistant h -order Bragg bands (photonic stop-bands) at the frequencies ω h determined by the condition where is the average refractive index. Obviously, away from the Bragg reflection bands, the periodic (ordered) structure is completely transparent, that is, transmission coefficient tends to unity at N →∞, which means zero extinction. Novel and unexpected effects are discovered when disorder is introduced to permittivity of the layers B ( Fig. 1b,d,e ). First, PhC stops being completely transparent outside the Bragg bands. Corresponding background extinction becomes non-zero. One can calculate it either within the rigorous phase formalism [7] , outlined in Methods, or from the following approximate recurrence relation for the transmission coefficient, , where the reflection coefficient describes the backscattering amplitude from the j -th layer B surrounded by the infinite barriers A, and | r j | ≪ 1. For the averaged logarithmic transmission, such approach leads to and This background extinction is clearly determined by uncompensated scattering on different layers B . The spectral dependence of equation (3) reflects the Fabry–Perot interference on the slab with the width w B . In addition to the Fabry–Perot scattering, our analysis reveals unexpected changes in the spectral amplitude and shape at the Bragg frequencies (1). From Fig. 1b , we observe that at the Bragg bands are no longer stop-bands. Depending on the values of σ B and the index h , the shape of the Bragg band changes drastically to a complete spectrum reversal, that is, it transforms from stop-band to pass-band. The shape of the Bragg band can be quite different depending on its location relative to the Fabry–Perot background (3). Next, we analyse how this Bragg band reversal depends on the magnitude and type of disorder. 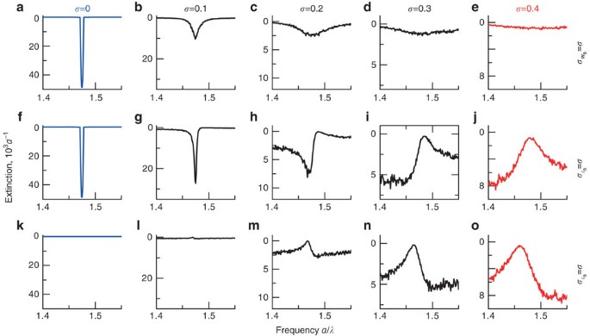Figure 2: Evolution of the Bragg bands for different types of disorder in the layer B. The averaged extinction spectra are shown in large scale in the proximity of fourth order Bragg band. (a–e)w-disorder. Thickness of layers A fluctuates around mean valuewith the dispersion. (f–j)ɛ-disorder. PermittivityɛBfluctuates around mean valuewith the dispersion,. (k–o)ɛ-disorder. PermittivityɛBfluctuates around mean value with the dispersion,(null contrast regime). Other parameters were as follows:ɛA=1.70,for (a–j) andfor (k–o),wB=0.38a,N=1,000,M=5,000. Figure 2 summarizes our numerical studies of different types of disorder. We consider the Bragg band with h =4. The slabs B are allowed to possess certain degrees of disorder, either in thickness ( for j -th layer with the mean value , referred to as w -disorder) or in permittivity ( for j -th layer with mean value , referred to as ɛ -disorder). The fluctuations are described by the normal distribution with dispersions and , respectively. Figure 2: Evolution of the Bragg bands for different types of disorder in the layer B. The averaged extinction spectra are shown in large scale in the proximity of fourth order Bragg band. ( a–e ) w -disorder. Thickness of layers A fluctuates around mean value with the dispersion . ( f – j ) ɛ -disorder. Permittivity ɛ B fluctuates around mean value with the dispersion , . ( k – o ) ɛ -disorder. Permittivity ɛ B fluctuates around mean value with the dispersion , (null contrast regime). Other parameters were as follows: ɛ A =1.70, for ( a – j ) and for ( k – o ), w B =0.38 a , N =1,000, M =5,000. Full size image We consider two different types of disorder, namely, w -disorder ( Fig. 2a–e ) and ɛ -disorder ( Fig. 2f–j ). We also examine specific photonic structure with permittivity of layers B fluctuating around the constant permittivity of layers A , lacking mean dielectric contrast, ( Fig. 2k–o ). The w -disorder leads to well-known degradation of Bragg band [17] , [18] , [19] , [23] , [32] , [33] , [34] , [35] , [36] ( Fig. 2a–e ). The key result of this work is presented in Fig. 2f–j : it is the transformation of the Bragg band in the spectra of 1D PhC with fluctuating dielectric constant and . The Bragg band shows an unexpected evolution with the strength of ɛ -disorder. First, the symmetric contour of Bragg band in the spectrum of ordered 1D PhC ( , Fig. 2f ) becomes asymmetric when weak disorder is introduced ( , Fig. 2g ). Next, further growth of the degree of disorder ( , Fig. 2h,i ) leads to an increasingly asymmetric shape of the spectrum. The turning point of the transformation is reversal of the band and conversion of the Bragg stop-band into a Bragg pass-band ( , Fig. 2j ). Thus, the photonic band structure of ɛ -disordered 1D PhC can be considered, in some sense, as inverted with respect to the photonic band structure of perfectly ordered 1D PhC; ordered 1D PhC is completely transparent in the whole spectral range except Bragg bands (photonic stop-bands), while ɛ -disordered 1D PhC is opaque outside the Bragg bands (photonic pass-bands). It is also instructive to consider 1D structure, where the permittivity of layers B still can fluctuate, but mean dielectric contrast is absent, . At the structure is spatially homogeneous and completely transparent, T ( ω )≡1. Disorder suppresses transmission and simultaneously reveals another effect: a pass-band arising at the Bragg frequency, and becoming more distinct with increase of disorder strength ( Fig. 2k–o ). The spectra of 1D PhC with ( Fig. 2f–j ) and spectra of 1D structure with ( Fig. 2k–o ) are radically different only for small disorder. At large disorder, when fluctuations in overcome the dielectric contrast , one gets the same result: pronounced Bragg pass-bands ( Fig. 2j,o ). To evaluate how departing from ideal Fano conditions would affect the results, we also calculated averaged extinction spectra as a function of ɛ -disorder degree in the layer A at fixed ɛ -disorder degree in the layer B , ( Fig. 3 ). First, the Fano peak becomes smaller when weak ɛ -disorder is introduced in the layer A ( , Fig. 3f ). Further growth of the degree of disorder ( and 0.15; Fig. 3g,h ) leads to complete degradation of the Fano peak. Second, the asymmetric Fano contour in the spectrum ( , Fig. 3i,m ) gradually becomes symmetric Bragg stop-band, when ɛ -disorder is increased in the layer A ( Fig. 3m–p ). Thus, the Fano resonance demonstrates strong survivability and unexpected condition should be achieved before the Fano signatures disappear completely. 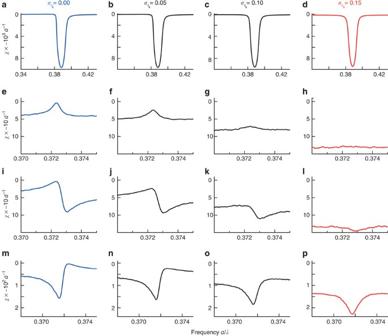Figure 3: Bragg bands of structures with disorder in the B layers as a function of disorder in the A layer. The averaged extinction spectra are shown in large scale in the proximity of fourth order Bragg band. (a–d) the spectrum with the dip (stop-band), (e–h) the spectrum with the peak (pass-band). (i–l) and (m–p) the two spectra with asymmetric profiles. Parameters of 1D PhC were,N=2000,M=5000.,ɛA=1.800,(a–d), 1.805 (e–h) 1.800 (i–l), 1.815 (m–p). Figure 3: Bragg bands of structures with disorder in the B layers as a function of disorder in the A layer. The averaged extinction spectra are shown in large scale in the proximity of fourth order Bragg band. ( a – d ) the spectrum with the dip (stop-band), ( e – h ) the spectrum with the peak (pass-band). ( i – l ) and ( m – p ) the two spectra with asymmetric profiles. Parameters of 1D PhC were , N =2000, M =5000. , ɛ A =1.800, ( a – d ), 1.805 ( e – h ) 1.800 ( i – l ), 1.815 ( m – p ). Full size image Localization and de-localization in disordered structures Here we will examine the correspondence between extinction spectra and light spatial distribution inside the PhC with ɛ -disorder ( Fig. 4 ). 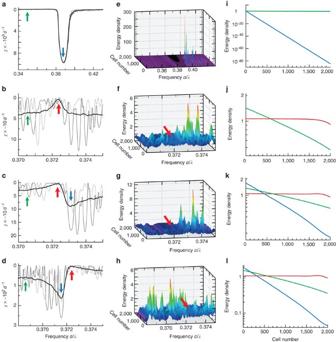Figure 4: De-localization of light at Bragg wavelength in 1D photonic crystals withɛ-disorder. (a–d) Averaged extinction spectraχ(λ) (thick curves) and extinction spectra for two realizations (thin curves) in the proximity of second order Bragg band. Arrow shows three regions: Fabry–Perot background (green), Bragg dip (blue) and Bragg peak (red). (e–h) Electromagnetic energy density distribution. Amplitude of fields normalized to the incident wave amplitude. (i–l) Averaged energy density logarithm distribution for the three spectral regions. Parameters of 1D PhC were,N=2,000,M=500.,ɛA=1.800,(a,e,i), 1.805 (b,f,j), 1.800 (c,g,k), 1.815 (d,h,i). Figure 4a–d demonstrates extinction spectra in the proximity of second order Bragg band in four cases with different spectral shape: Bragg stop-band ( Fig. 4a ), Bragg pass-band ( Fig. 4b ) and two intermediate cases with spectra related by mirror symmetry, with respect to the Bragg frequency ( Fig. 4c,d ). For each case, we present averaged extinction spectra and also the spectra for two given disorder realizations. It is important, that the spectra for individual random realizations look always generally similar to the averaged extinction spectra ( Fig. 4a–d ), although they consist of a number of dips originating from spatially localized eigenmodes. This is a manifestation of the structure ergodicity that is the extinction self-averaging for large number of layers N . Our previous analysis of Figs 1 and 2 allows to distinguish between three qualitatively different regions in optical spectra. We will term them as Fabry–Perot background (green arrow in Fig. 4 ), Bragg dip (pass-band with large T and small χ , blue arrow) and Bragg peak (stop-band with small T and large χ , red arrow). Figure 4b–d shows that the Bragg pass-band is always present for individual disorder realizations and for averaged extinction spectra as well. The amplitude of extinction fluctuations is substantially quenched in the pass-band region, and the extinction itself tends to zero. Outside the Bragg pass-band region, the amplitude of fluctuations is large both for Fabry–Perot and for Bragg dip ( Fig. 4d ). Figure 4: De-localization of light at Bragg wavelength in 1D photonic crystals with ɛ -disorder. ( a – d ) Averaged extinction spectra χ ( λ ) (thick curves) and extinction spectra for two realizations (thin curves) in the proximity of second order Bragg band. Arrow shows three regions: Fabry–Perot background (green), Bragg dip (blue) and Bragg peak (red). ( e – h ) Electromagnetic energy density distribution. Amplitude of fields normalized to the incident wave amplitude. ( i – l ) Averaged energy density logarithm distribution for the three spectral regions. Parameters of 1D PhC were , N =2,000, M =500. , ɛ A =1.800, ( a , e , i ), 1.805 ( b , f , j ), 1.800 ( c , g , k ), 1.815 ( d , h , i ). Full size image Figure 4e–h presents electromagnetic field energy density distribution along 1D structure at different frequencies for a given disorder realization. Pronounced peaks correspond to different localized modes. Figure 4f–h demonstrates almost complete absence of the localized states in the spectral range of Bragg pass-band. On the other hand, outside the Bragg pass-band, the light is strongly localized, in accordance with Fig. 4b–d . Because extinction equals the inverse localization length, strong localization means large extinction. The same results follow from Fig. 4i–l , presenting the averaged energy density of electromagnetic field along the structure in logarithmic scale. In the pass-band region, the energy density is homogeneously distributed, excepting structure boundaries, while in the spectral range of FabryPerot background and Bragg stop-band, it exponentially decays along the structure. The slope of the curves in Fig. 4i–l corresponds to inverse localization length. To summarize, Fig. 4 clearly demonstrates light de-localization taking place at Bragg frequency in 1D PhC with ɛ -disorder. 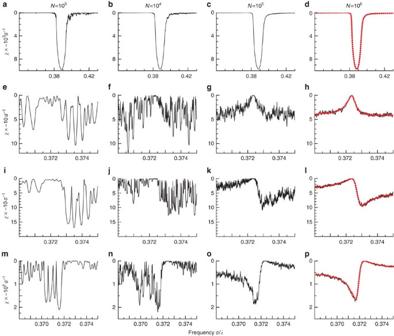Figure 5: Demonstration of ergodicity of the 1D disordered structures. Extinction spectra of one single structure realization as a function of the sample lengthN. (a–d) the spectrum with the dip, (e–h) the spectrum with the peak. (i–l) and (m–p) the two spectra with asymmetric profiles. The sample parameters were,,ɛA=1.800,(a–d), 1.805 (e–h), 1.800 (i–l), 1.815 (m–p). The red-dotted curves are extinction spectra averaged over an ensemble of 103realizations of samples of 104unit cells in lengths. Figure 5 demonstrates the ergodic self-averaging behaviour of the Fano extinction spectrum with the structure length. An extinction spectrum of a single realization of a long enough disordered structure is tending to the extinction spectrum of short structure averaged over big enough ensembles of different realization (shown in Fig. 5 by red-dotted curve). Figure 5: Demonstration of ergodicity of the 1D disordered structures. Extinction spectra of one single structure realization as a function of the sample length N . ( a – d ) the spectrum with the dip, ( e – h ) the spectrum with the peak. ( i – l ) and ( m – p ) the two spectra with asymmetric profiles. The sample parameters were , , ɛ A =1.800, ( a – d ), 1.805 ( e – h ), 1.800 ( i – l ), 1.815 ( m – p ). The red-dotted curves are extinction spectra averaged over an ensemble of 10 3 realizations of samples of 10 4 unit cells in lengths. Full size image Analytical model To clarify the origin of the effects revealed by the numerical simulation, we have developed a theoretical model. We have used the phase formalism [7] applicable to arbitrary 1D systems. Starting directly from the transfer matrix method [15] , we have determined the extinction χ from the Fokker-Planck equations for the distribution of the electric field phase. Below, we discuss the main results of the theory; more details are given in Methods. We focus on the spectral range close to the given Bragg frequency ω h (1) and assume weak dielectric contrast. These two conditions are already sufficient to reproduce the results of numerical simulation analytically. Compact closed form for extinction can be obtained under two additional conditions: strong enough disorder as compared with the average value of the dielectric contrast, , and thickness of the layers B larger than the light wavelength, that is, . Here we have introduced the average phase incursion Φ h in the layers B at the Bragg resonance. This phase Φ h is the key parameter of the problem. Under the above assumptions, the extinction reduces to the Fano function of the dimensionless frequency Ω=( ω − ω h )/Γ h and the Fano parameter The relative resonance width Γ h / ω h is given by . Expression of type (4) was first obtained by Fano to describe asymmetric lines in auto-ionization spectra [12] . Later, Fano formalism was successfully applied for interpretation of characteristic spectral features of various objects [14] , [37] , [38] , [39] , [40] , [41] , [42] , including 3D PhC – synthetic opals. [22] The Fano asymmetry parameter q governs the spectral shape. Its value is determined by the specific parameters of the object under consideration, in our case, it is given by equation (5) and depends on the phase incursion Φ h . Let us now analyse equation (4) and compare it with the numerical simulation. Far from the Bragg condition, that is, at Ω ≫ q , extinction (4) reduces to . This is just the background extinction (3), revealed in . As equation (4) was derived in the Bragg resonance vicinity, it neglects frequency dependence of the background (3). Near to the Bragg frequency (1), corresponding to Ω=0, the localization length can either increase or decrease, as described by the Fano spectrum (4). A general explanation of this effect is the interference between the single-scattering events, determining the broad Fabry–Perot background, and coherent multiple scattering, essential near the Bragg resonance. The crucial condition for this interference is the absence of w -disorder, in agreement with Fig. 2 . The microscopic origin of the enhancement (stop-band) and suppression (pass-band) of localization at the Bragg wavelength is rather subtle. The analysis becomes most simple when the mean contrast vanishes, and the Fano parameter reads just q =−cotΦ h . Two cases can be then separated. In the first case, cosΦ h =0, that is, w B / a =(2 k +1)/(2 h ), k =0,1.... Then it turns out, that at the Bragg frequency ω h , the nodes of the electric field are centred at the layers B . This wave is insensitive to the fluctuations of and does not decay (Bragg pass-band), that is, q =0 and χ (Ω=0)=0, in agreement with equation (4). This can be interpreted as Borrmann effect generalized for disordered system. Conventional Borrmann effect is the enhancement of transmission for periodic absorbing structures [43] , [44] at the stop-band edge. Similar localization suppression near the band gap is quite known for disordered 1D systems. [6] , [7] , [8] , [9] In the second case, sinΦ h =0, that is, w B / a = k / h , k =1,2,... Then, the linear in contrast contribution to the reflection coefficient of the single layer r j (2) vanishes and the second order term becomes important. It is crucial that the averaged value of this term is non-zero, that is, average amplitude reflection coefficient is the same for all layers. Constructive interference of reflected waves leads to the peak in the extinction χ ( ω ), in agreement with equation (4). This is a rather unconventional disorder-induced Bragg stop-band, determined by the fluctuations of the permittivity . Arbitrary values of the phase Φ h correspond to the Fano profile (4), determined by the interplay of the Borrmann effect-related pass-band and the disorder-induced Bragg stop band. The Fano regime holds provided that the thickness of the layers B is on the order of the light wavelength. At very large and very small values of w B / λ the interference should be not relevant. Large values of w B / λ correspond to the regime of geometrical optics. It is realized for sufficiently high-order h of the Bragg bands. The relative width of the Bragg band Γ h / ω h grows with h . At large h , the Bragg band linewidth becomes comparable with the interband distances, so that different Fano resonances overlap and smear out. The opposite case of thin layers B , w B ≪ λ is instructive as well. It is similar to the Rayleigh scattering regime for 1D systems. To this end, the second order in contrast term in the B -layer reflectivity r j can be neglected. Thus, the disorder-induced contrast is quenched and the extinction is solely determined by the Borrmann effect, leading to the dip in χ ( ω ) (pass-band). When average dielectric contrast is present, , the results above remain qualitatively the same. In the Fano regime ( wB ∼ λ ) dielectric contrast affects the value of the Fano parameter. One can see from equation (4), that for very large contrast, the parameter q also becomes large, leading to the peak in extinction and to the Bragg stop-band. However, equation (4) is valid only provided that the average dielectric contrast is not large as compared with disorder. In the Rayleigh regime ( w B ≪ λ ), the extinction spectrum has a Bragg maximum with a dip due to the Borrmann effect at the edge. These results can be summarized as follows (see also Table 1) : for small thicknesses of the layers B (Rayleigh scattering regime), extinction spectrum has a narrow pass-band originating from the Borrmann effect and, for non-zero average contrast, an additional Bragg stop-band. For the thicknesses comparable to the light wavelength (Fabry–Perot regime), the Fano-like extinction strongly depends on the ratio w B / λ , which is caused by the interplay of the Borrmann effect and the disorder-induced contrast. Finally, for the large thicknesses (geometrical optics), the Fano feature is smeared out. Such transition from the Rayleigh scattering regime to the geometrical optics has been discussed for photonic crystals already in the original paper of S. John [45] , our findings demonstrate the Fano interference in the intermediate case. Table 1 Regimes of light propagation in ɛ -disordered photonic crystals for different thicknesses of layers B . Full size table Thus, our theory allows to interpret the features in Figs 1 , 2 , 3 , 4 , 5 as Fano resonances. To provide further justification of this result, we have fitted calculated extinction spectra by original Fano formula [12] to extract the Fano asymmetry parameter q . The most remarkable results were obtained processing the dependence of the spectra on the relative thickness w B / a of the layers B ( Fig. 6a ). Figures 6b–d present q -parameters extracted from numerical spectra in Fig. 6a for first, second and third order Bragg bands ( h =1,2,3) and the theoretical expression (5). One can see an excellent agreement between numerical and analytical results. Substantial deviation from the Fano regime is present only for the first order Bragg band, when the value of w B / a is small, and is consistent with the Rayleigh regime discussed above. The shape of the Bragg bands is strictly periodically transformed with variation of w B , complete cycles can be observed. Each cycle includes the following sequence: symmetric stop-band ( q →−∞), corresponding to the maximum of the sin-like Fabry–Perot background; asymmetric line with flat long-wavelength wing and steep short-wavelength wing ( q <0); symmetric pass-band ( q =0); asymmetric line with flat short-wavelength wing and steep long-wavelength wing ( q >0); again symmetric stop-band ( q →∞). This is the scanning of the Bragg band by the sin-like Fabry–Perot contour equation (3) and is quite similar to the q -reversal of the Fano resonance in atomic systems for Rydberg lines interacting with the continuum with energy-dependent phase [13] . When w B / a changes from zero to unity, h periods of the background pass through the h -order Bragg maximum, which demonstrates h full cycles of the shape transformation, in complete agreement with equation (5). 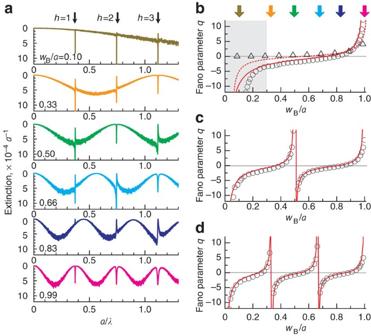Figure 6: Bragg band transformation and Fano parameter in 1D photonic structure withɛ-disorder as a function of the layer A thickness. (a) Averaged extinction spectra ofɛ-disordered 1D PhC with variation of thickness of B layerswB/a. (b–d) Fano parameterqfor first order Bragg band (b), second order (c) and third order Bragg band (d). Lines and symbols present Fano parameterq, calculated by equation (4) and extracted from numerical spectra, respectively. Arrows on top of panel (b) show the values of the parameterwB/afor the spectra shown in panel (a). Calculation was performed for the following values of parameters:ɛA=1.80,,,N=2,000,M=1,000. Triangles and dashed lines on panel (b) correspond to the case of zero average dielectric contrast,. Shaded area on panel (b) marks Rayleigh regime. Figure 6: Bragg band transformation and Fano parameter in 1D photonic structure with ɛ -disorder as a function of the layer A thickness. ( a ) Averaged extinction spectra of ɛ -disordered 1D PhC with variation of thickness of B layers w B / a . ( b – d ) Fano parameter q for first order Bragg band ( b ), second order ( c ) and third order Bragg band ( d ). Lines and symbols present Fano parameter q , calculated by equation (4) and extracted from numerical spectra, respectively. Arrows on top of panel ( b ) show the values of the parameter w B / a for the spectra shown in panel ( a ). Calculation was performed for the following values of parameters: ɛ A =1.80, , , N =2,000, M =1,000. Triangles and dashed lines on panel ( b ) correspond to the case of zero average dielectric contrast, . Shaded area on panel ( b ) marks Rayleigh regime. Full size image Our analytical and numerical results provide new insight into light localization and de-localization phenomena in random media. We demonstrate that, even in the simplest possible and (seemingly) thoroughly studied and well-known 1D layered dielectric structure, the picture of light localization and de-localization is much richer than was suggested before. The qualitative difference between the geometric ( w ) and compositional ( ɛ ) disorder has been demonstrated; to the best of our knowledge it has never been analysed in detail up to now. Our results explain how Bragg bands can transform from the well-known stop-band to the discovered pass-band, that is, from light localization to light de-localization. The origin of the unique transmutability of the Bragg band is the interference between Bragg multiple scattering and disorder-induced Fabry–Perot single-scattering. We have demonstrated that this interference can be described within the Fano approach, which allowed us to find the cyclic dependence of the line shape on the layer thickness w B . This Fano resonance, where one of the scattering channels is random, has been theoretically described for the first time. The random nature of the channel does not destroy the bright interference phenomena in optical spectra. This Fano resonance and Anderson localization phenomenon share the same physical origin, namely, the interference between different paths, arising from multiple scattering of the photons by the structure imperfections. This general nature of the effect provides the possibility of its manifestation in various systems, not limited to the electromagnetic problems. For instance, disorder-Fano resonance should be also present in the binary semiconductor superlattice, where the effective carrier masses in one of the components fluctuate from layer to layer. We show in Methods how the Schrödinger equation for this system can be exactly mapped to the Maxwell equation for wave propagation in the random dielectric stack, which unifies electron and photon problems. Similar features should be also manifested in phonon transport through superlattices with compositional disorder. Semiconductor heterostructures are very promising for the controllable study of the effect, because quantum cascade lasers with more than a thousand layers [46] , [47] , as well as deterministic aperiodic photonic structures with hundreds of layers, are efficiently grown nowadays [48] , [49] . Observation of very similar Fano resonances in opals [22] calls for future theoretical analysis and hints that some of the effects studied here may unexpectedly survive even in 3D, even though localization phenomena in 1D and 3D systems are generally quite different. [30] We believe that the effects discovered in the present study, including the impressive Fano transformation of the Bragg bands, conversion of the localized states into the delocalized states and vice versa, should occur in other systems, including dielectric photonic structures, semiconductor superlattices with effective mass disorder, and in a variety of other disordered systems with proper fluctuations of the response of one of the periodically repeating components. The current study paves a way for tailoring disordered structures with the localization absent for Bragg wavelengths. A further search for different systems with the extraordinary transmission of photons, as well as electrons, can substantially increase the applicability range of our results. Calculation of the extinction We first utilize the smooth envelope technique in low-contrast approximation. Within each j -th layer A , electric field can be written as where . Near the Bragg condition equation (1), the amplitudes U and V in equation (6) can be presented as a product of the slow-varying envelopes u and v , multiplied by the rapidly changing exponential factors, U j = u ( j )(−1) jh and V j = v ( j )(−1) jh . After that, we write the transfer matrix through the layer j up to the second order in dielectric contrast. This transfer matrix is equivalent to the following system of differential equations for smooth envelopes of forth- and back-propagating waves: where The phase Φ h can we written as Φ h =π bh /( a + b ), and is the dimensionless dielectric contrast. It follows from equation (7) that the function α( j ) describes the local phase incursion, and the function β ( j ), determined by the dielectric contrast, describes the scattering of the waves. Both these quantities are random. Langevin-type equation (7) describe the wave dynamics under the influence of the random force η ( j ). The localization length 1/ χ is formally given by . The standard procedure to determine the value of χ is to reduce the Langevin equations to the Fokker-Planck one. [7] This is not trivial because of the non-Gaussian statistics of the η 2 term in equation (7). This term has the crucial role in our consideration. For instance, in ref. 20 , this term has not been taken into account, so our Fano result (4) cannot be reproduced. The analytical results of ref. 21 have been obtained including the quadratic terms but only in random-phase approximation, which is not sufficient for considered system. In our case, we have replaced η 2 in equation (7) by its value, averaged over disorder, ignoring the higher order correlators. After that, the problem can be solved by the standard techniques of ref. 7 . The general result for the extinction can be then presented as (see also ref. 21 ) where the phase ψ is determined from exp( i ψ )= i exp(− i Φ h )/ u / v , δβ = β −〈 β 〉 and δα = α −〈 α 〉. It satisfies the Langevin equation following from equation (8). At such frequencies, that 〈α〉 ≫ β , the phase ψ is homogeneously distributed over the interval [0,...2 π ]. Only the second term in equation (9) is then non-zero, leading to equation (3). Otherwise, one should obtain the distribution function F of the phase ψ from the Fokker–Planck equation, corresponding to equation (10): Approximate solution of equation (11) for Φ h ≫ 1 reads and, after averaging in equation (9), yields equation (4). Here Ω and q are dimensionless frequency and the Fano parameter, defined after equation (4). Photonic and electronic problems The transfer matrices for given slab w B with dielectric constant ɛ B reads [28] where wavevector , and the basis is electric field E ( z ) and its derivative . On the other hand, electron transmission matrix through a layer with constant potential U B and effective mass m B is where and the basis is wavefunction and its scaled derivative m B /( m A k B ) dψ / dz . Here m A and U A are effective mass and potential in the layers A , used a a reference. Comparing equations (13) and (14), we see that the fluctuations of the effective mass m B exactly correspond to the ɛ -disorder in PhC. How to cite this article: Poddubny, A. N. et al . Fano interference governs wave transport in disordered systems. Nat. Commun. 3:914 doi: 10.1038/ncomms1924 (2012).